Homeostatic control of polo-like kinase-1 engenders non-genetic heterogeneity in G2 checkpoint fidelity and timing The G2 checkpoint monitors DNA damage, preventing mitotic entry until the damage can be resolved. The mechanisms controlling checkpoint recovery are unclear. Here, we identify non-genetic heterogeneity in the fidelity and timing of damage-induced G2 checkpoint enforcement in individual cells from the same population. Single-cell fluorescence imaging reveals that individual damaged cells experience varying durations of G2 arrest, and recover with varying levels of remaining checkpoint signal or DNA damage. A gating mechanism dependent on polo-like kinase-1 (PLK1) activity underlies this heterogeneity. PLK1 activity continually accumulates from initial levels in G2-arrested cells, at a rate inversely correlated to checkpoint activation, until it reaches a threshold allowing mitotic entry regardless of remaining checkpoint signal or DNA damage. Thus, homeostatic control of PLK1 by the dynamic opposition between checkpoint signalling and pro-mitotic activities heterogeneously enforces the G2 checkpoint in each individual cell, with implications for cancer pathogenesis and therapy. The presence of lesions such as DNA double-strand breaks (DSBs) triggers activation of a cell cycle checkpoint mechanism during the G2 phase of the cell cycle (‘the G2 checkpoint’), which acts to prevent mitotic entry. The molecular components of the G2 checkpoint machinery have been extensively characterized [1] , [2] , [3] , [4] , and include proteins that sense DSBs [5] , [6] , signal their presence via a kinase-dependent catalytic cascade [7] , [8] , [9] and enforce G2 arrest [10] , [11] , [12] , [13] . Despite intensive study, however, the mechanisms that control checkpoint recovery and progression into mitosis after G2 arrest remain unclear. Ensemble studies on cell populations suggest that G2 checkpoint activation by DNA damage arrests mitotic entry until DNA repair allows checkpoint signalling to fall below a defined threshold. It was initially believed that G2 checkpoint recovery could occur only after the complete resolution of all DNA damage, but studies on radiation-induced G2 arrest in mammalian cells showed that cells could recover without fully resolving DNA lesions [14] . This was at first attributed to ‘checkpoint adaptation’ [15] , a phenomenon initially described in budding yeast [16] , [17] , wherein cells become desensitized to checkpoint signalling after prolonged G2 arrest induced by irreparable DSBs. However, later studies have refuted this hypothesis, suggesting instead that the G2 checkpoint in mammalian cells cannot be activated by small amounts of DNA damage [18] , but only triggers G2 arrest when the amount of damage is above a defined threshold [19] , [20] , estimated, for instance, to be ~20 DSBs in human fibroblasts. Ensemble studies also suggest that checkpoint signalling acts as an ‘on-off’ switch to ablate pro-mitotic signals, such as the activity of the pro-mitotic kinases polo-like kinase-1 (PLK1) or CDK1-Cyclin B1, when cells are arrested in G2. Such a switch is proposed to work through several routes. For instance, G2 checkpoint activation by DNA damage causes dephosphorylation [21] , [22] as well as degradation of PLK1 (ref. 23 ). Moreover, it triggers the inhibition of Cyclin B1 synthesis and nuclear localization [24] , [25] , [26] , [27] . These checkpoint-initiated processes are believed to ablate pro-mitotic activities until the ongoing repair of DNA damage allows checkpoint signalling to fall below a threshold, allowing the activation of pro-mitotic enzymes, and entry into mitosis [19] , [28] . On the other hand, pro-mitotic activities have also been implicated in silencing checkpoint activity [29] , [30] , suggesting a complex regulatory process involving feedback between checkpoint enforcement and pro-mitotic activities. However, ensemble studies typically report average cell behaviour, masking variations at the single-cell level that are critical to decisions that determine cellular outcome [31] , [32] . Moreover, single-cell studies tracking live cells allow correlations to be drawn over time between individual cellular outcomes and molecular events [33] , exposing previously unrecognized intrinsic or extrinsic factors affecting the decisions that determine outcome [34] , [35] . To address these issues, we have studied G2 checkpoint recovery and mitotic entry in single cells exposed to double-strand DNA breakage. Unexpectedly, our findings suggest that at the level of single cells there is neither a well-defined fixed threshold of checkpoint activation signal or underlying DNA damage below which checkpoint recovery proceeds, nor that the G2 checkpoint acts as an ‘on-off’ switch to ablate pro-mitotic signals when it is active in G2-arrested cells. Instead, we observe using several different experimental systems that single cells heterogeneously recover from G2 arrest with varying levels of checkpoint activation signal or DNA damage, in a manner correlated with the duration of arrest. We demonstrate that this heterogeneity in G2 checkpoint outcome is controlled via PLK1. PLK1 activity measured by a fluorescent reporter is not switched off in G2-arrested cells, but instead, continually accumulates from its initial level. In each cell, the rate of accumulation is inversely correlated with the level of checkpoint activation. Individual cells remain arrested in G2 for different periods until cumulative PLK1 activity reaches a critical threshold, which gates mitotic entry. When this occurs, cells recover from G2 arrest and enter mitosis, regardless of the level of residual DNA damage. Thus, single-cell measurements reveal considerable heterogeneity in the fidelity and timing of G2 checkpoint enforcement, which is not genetically determined in that it manifests in individual cells from the same population. Instead, our findings suggest a new model wherein PLK1 activity integrates the dynamic opposition between checkpoint signalling and pro-mitotic activities in single cells, triggering non-genetic heterogeneity in the outcome of G2 checkpoint activation in each cell. Non-genetic heterogeneity in G2 checkpoint recovery We used two distinct experimental methods to test whether individual cells in the same population recover from damage-induced G2 arrest and enter mitosis when checkpoint signalling falls below a threshold marking a set amount of residual DNA damage. First, we measured the number of nuclear foci containing the phosphorylated form of histone H2AX (γH2AX), a robust and widely used marker for the presence of DSBs [36] , in single cells that had escaped damage-induced G2 arrest and entered prometaphase ( Fig. 1a ). Second, we followed by time-lapse imaging the formation of foci by a green fluorescent protein (GFP)-tagged form of MDC1, a protein whose rapid recruitment to sites of DNA damage correlates with G2 checkpoint activation [37] , [38] , in living single cells undergoing damage-induced G2 checkpoint arrest and recovery ( Fig. 2a ). 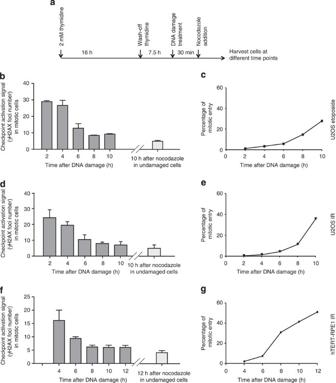Figure 1: Cells enter mitosis with variable numbers ofγH2AX foci after DNA damage. (a) The experimental protocol. U2OS cells were synchronized in G2 by thymidine block before exposure to DNA damage (either a brief pulse of etoposide or ionizing radiation, as indicated in the text). Synchronized, damaged cells were treated with nocodazole 30 min later to trap in mitosis cells that had recovered from G2 arrest, before staining for phospho-histone H3 (pH3) and γH2AX. (b) The bar chart plots the average level of checkpoint activation signal, denoted by γH2AX foci number, in U2OS cells that had recovered from G2 arrest and entered mitosis at different time points after etoposide exposure. The average number of mitotic γH2AX foci in undamaged cells arrested in nocodazole for 10 h is shown as control. (c) The chart plots the average percentage of U2OS cells that entered mitosis at different time points after etoposide exposure. (d) The bar chart plots the average level of checkpoint activation signal, denoted by γH2AX foci number, in U2OS cells that had recovered from G2 arrest and entered mitosis at different time points after 1.5 Gy IR treatment. The average number of mitotic γH2AX foci in undamaged cells arrested in nocodazole for 10 h is shown as a control. (e) The chart plots the average percentage of U2OS cells that entered mitosis at different time points after 1.5 Gy IR treatment. (f) RPE1 cells synchronized by thymidine block were exposed to 1 Gy IR, and treated as ina. The bar chart shows the average level of checkpoint activation signal (γH2AX foci) in cells that had recovered from G2 arrest and entered mitosis at different time points after damage exposure. The average number of mitotic γH2AX foci in undamaged cells arrested in nocodazole for 12 h is shown as a control. (g) The chart plots the average percentage of RPE1 cells that entered mitosis at different time points after 1 Gy IR treatment. The experiments in all panels were run in triplicate. Charts depict the mean and s.e.m. Figure 1: Cells enter mitosis with variable numbers of γ H2AX foci after DNA damage. ( a ) The experimental protocol. U2OS cells were synchronized in G2 by thymidine block before exposure to DNA damage (either a brief pulse of etoposide or ionizing radiation, as indicated in the text). Synchronized, damaged cells were treated with nocodazole 30 min later to trap in mitosis cells that had recovered from G2 arrest, before staining for phospho-histone H3 (pH3) and γH2AX. ( b ) The bar chart plots the average level of checkpoint activation signal, denoted by γH2AX foci number, in U2OS cells that had recovered from G2 arrest and entered mitosis at different time points after etoposide exposure. The average number of mitotic γH2AX foci in undamaged cells arrested in nocodazole for 10 h is shown as control. ( c ) The chart plots the average percentage of U2OS cells that entered mitosis at different time points after etoposide exposure. ( d ) The bar chart plots the average level of checkpoint activation signal, denoted by γH2AX foci number, in U2OS cells that had recovered from G2 arrest and entered mitosis at different time points after 1.5 Gy IR treatment. The average number of mitotic γH2AX foci in undamaged cells arrested in nocodazole for 10 h is shown as a control. ( e ) The chart plots the average percentage of U2OS cells that entered mitosis at different time points after 1.5 Gy IR treatment. ( f ) RPE1 cells synchronized by thymidine block were exposed to 1 Gy IR, and treated as in a . The bar chart shows the average level of checkpoint activation signal (γH2AX foci) in cells that had recovered from G2 arrest and entered mitosis at different time points after damage exposure. The average number of mitotic γH2AX foci in undamaged cells arrested in nocodazole for 12 h is shown as a control. ( g ) The chart plots the average percentage of RPE1 cells that entered mitosis at different time points after 1 Gy IR treatment. The experiments in all panels were run in triplicate. Charts depict the mean and s.e.m. 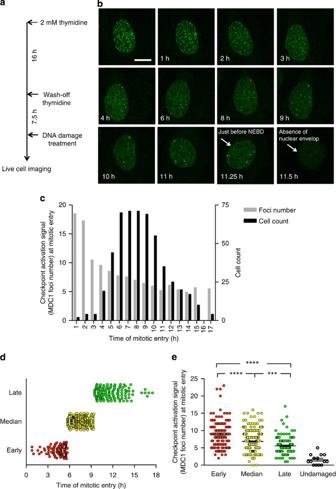Figure 2: Cells enter mitosis with variable numbers of MDC1 foci after DNA damage in live cell imaging. (a) The experimental protocol. U2OS cells were synchronized in G2 by thymidine block before exposure to a brief pulse of etoposide. Synchronized, damaged cells were subjected to live cell imaging to monitor damage foci. (b) Serial imaging of U2OS cells expressing MDC1-GFP following exposure to etoposide. Serial images were analysed to identify the first image exhibiting visible dissipation of nuclear fluorescence marking absence of the nuclear envelope (final panel, 11.5 h). MDC1-GFP foci number was enumerated just before nuclear envelope breakdown (NEBD) at mitotic entry, 15 min before this event (penultimate panel, 11.25 h). Experimental procedures were as described ina. Images are representative of multiple independent experiments. Scale bar, 5 μm. (c) The graph depicts the level of checkpoint activation signal, denoted by MDC1 foci number (yaxis), retained in cells just before NEBD at mitotic entry, against the time taken to reach NEBD after damage exposure (xaxis). The grey bars show the distribution of average retained foci number in cells undergoing NEBD each hour and the black bars show the total number of cells undergo NEBD each hour. (d) Cells depicted incwere grouped into three categories based on the time taken to enter mitosis after DNA damage. Cells that entered mitosis early (1st quartile, red) were compared with those entering around the median (2nd and 3rd quartiles, yellow) or late (4th quartile, green). The early and late categories were selected to include equal cell numbers. (e) Displays the statistical significance of differences in the foci number between the three categories using the analysis of variance/Bonferroni test. Notably, the remaining level of MDC1 foci number at mitotic entry in the three categories of damage-exposed cells is also significantly higher than that from cells without DNA damage treatment (white). The mean (bar) and s.e.m. (whiskers) are shown (***P<0.0001; ****P<0.00001). Full size image Figure 2: Cells enter mitosis with variable numbers of MDC1 foci after DNA damage in live cell imaging. ( a ) The experimental protocol. U2OS cells were synchronized in G2 by thymidine block before exposure to a brief pulse of etoposide. Synchronized, damaged cells were subjected to live cell imaging to monitor damage foci. ( b ) Serial imaging of U2OS cells expressing MDC1-GFP following exposure to etoposide. Serial images were analysed to identify the first image exhibiting visible dissipation of nuclear fluorescence marking absence of the nuclear envelope (final panel, 11.5 h). MDC1-GFP foci number was enumerated just before nuclear envelope breakdown (NEBD) at mitotic entry, 15 min before this event (penultimate panel, 11.25 h). Experimental procedures were as described in a . Images are representative of multiple independent experiments. Scale bar, 5 μm. ( c ) The graph depicts the level of checkpoint activation signal, denoted by MDC1 foci number ( y axis), retained in cells just before NEBD at mitotic entry, against the time taken to reach NEBD after damage exposure ( x axis). The grey bars show the distribution of average retained foci number in cells undergoing NEBD each hour and the black bars show the total number of cells undergo NEBD each hour. ( d ) Cells depicted in c were grouped into three categories based on the time taken to enter mitosis after DNA damage. Cells that entered mitosis early (1st quartile, red) were compared with those entering around the median (2nd and 3rd quartiles, yellow) or late (4th quartile, green). The early and late categories were selected to include equal cell numbers. ( e ) Displays the statistical significance of differences in the foci number between the three categories using the analysis of variance/Bonferroni test. Notably, the remaining level of MDC1 foci number at mitotic entry in the three categories of damage-exposed cells is also significantly higher than that from cells without DNA damage treatment (white). The mean (bar) and s.e.m. (whiskers) are shown (*** P <0.0001; **** P <0.00001). Full size image Several lines of evidence substantiate that the enumeration of γH2AX foci in mitotic cells can be used as a surrogate measurement for signals that maintain checkpoint arrest (hereafter termed the ‘checkpoint activation signal’) during G2 checkpoint recovery. γH2AX foci formation marks the presence of DSBs [36] or structural aberrations in chromatin [39] , or, when induced by genetic means, can activate the G2 checkpoint even in the absence of DNA damage [40] , [41] . We find that the kinetics of γH2AX foci formation correlates with the activation of PIKK-family kinases like ATM and ATR, essential mediators of the G2 checkpoint signalling [42] ( Supplementary Fig. 1A–C ). Finally, when the phosphatases responsible for removing γH2AX phosphorylation are inactivated, γH2AX foci persist after the completion of DSB repair; as a result, cell cycle arrest also persists [41] , [43] . As per the experimental design shown in Fig. 1a , U2OS cells synchronized in the G2 phase (indicated by 4N DNA content, and the low percentage of mitotic cells marked by high phospho-histone H3 staining, Supplementary Fig. 1D ) were treated with 10 μM etoposide for 8 min. Nocodazole was added 30 min later to trap cells in mitosis after exit from G2 arrest, followed by enumeration of γH2AX foci ( Supplementary Fig. 1E ). Because DNA repair largely ceases upon mitotic entry [44] leaving unrepaired DNA damage sites marked by early checkpoint components, such as γH2AX foci or MDC1 (ref. 45 ), the measurement of γH2AX in cells trapped in prometaphase reflects the level of checkpoint activation signal at the time of G2 checkpoint recovery and exit. Figure 1b shows the residual checkpoint activation signal (γH2AX foci number) over time for single U2OS cells that entered mitosis after DNA damage-induced G2 arrest, and in Fig. 1c , the proportion of cells entering mitosis following recovery from G2 arrest. The checkpoint activation signal is elevated at all time points in etoposide-treated cells compared with undamaged controls ( Fig. 1b ), in the short duration of the nocodazole-induced mitotic trap ( Supplementary Fig. 1F ), speaking against the de novo formation of γH2AX foci as a result of mitotic arrest in this experimental setup [46] , [47] , [48] . Surprisingly, however, cells which recover from G2 arrest to enter mitosis at earlier time points, do so with a higher level of checkpoint activation signal than do cells whose G2 checkpoint recovery occurs later. A similar correlation was evident ( Fig. 1d, e ) in cells that had been treated with a dose (1.5 Gy) of ionizing radiation (IR) calibrated ( Supplementary Fig. 1G , H) to elicit a similar level of checkpoint activation signal as the etoposide treatment used in the preceding experiments. We performed metaphase spreads to test whether cells that recover from G2 arrest and enter mitosis bearing γH2AX foci harbour unrepaired DNA breakage. Indeed, we observed an elevated level of metaphase breaks in cells that entered mitosis after DNA damage treatment ( Supplementary Fig. 1I ). The mean number of chromosome breaks per cell corresponds to the mean level of observed γH2AX foci in prometaphase cells, albeit with high variance given that one metaphase break may correspond to ~10–20 γH2AX foci [19] . A similar correlation is evident in immortalized but non-transformed hTERT-RPE1 cells treated in the same way ( Fig. 1f, g and Supplementary Fig. 1J ), suggesting that our results are neither cell type specific nor simply a feature of cancer cell lines alone. Time-lapse imaging ( Fig. 2a ) using GFP-tagged MDC1, a marker correlated with G2 checkpoint activation [37] , [38] , yields a similar result. Notably, time-lapse imaging permits visualization of MDC1-GFP foci at the time of recovery from G2 arrest (rather than later in prometaphase using γH2AX foci in the preceding experiments). U2OS cells expressing MDC1-GFP were synchronized in G2, and MDC1-GFP foci were enumerated from exposure to etoposide-induced damage until mitotic entry denoted by nuclear envelope break down (NEBD; Fig. 2b ). Cells recovering from G2 arrest were grouped based on the timing of mitotic entry into three categories (early, representing the 1st quartile of the distribution; median, the 2nd and 3rd quartiles; late, the 4th quartile). Again, live cell imaging shows that cells in the early category recover with a higher level of the checkpoint activation signal than those in the median or late categories ( Fig. 2c–e ). The number of MDC1-GFP foci measured at mitotic entry diminished over time and eventually reached an average around six foci per cell ( Fig. 2c ). This value is slightly lower than the plateau value of γH2AX foci measured in mitosis, but significantly higher than the background in undamaged cells ( Fig. 2d,e ). Thus, collectively, our observations demonstrate that cells recovering from damage-induced G2 arrest enter mitosis with varying levels of checkpoint activation signal, in a manner that is dependent on the duration of G2 arrest. This is inconsistent with current models of the G2 checkpoint, which predicate that cells recover from G2 arrest when the checkpoint activation signal reaches a negligible level or falls below a well-defined threshold. Moreover, the broad distribution of residual checkpoint activation signal that is detected in mitotic cells, and its evident time correlation, demonstrates the existence of significant heterogeneity at the level of single cells from the same population. Neither this non-genetic heterogeneity nor the mechanisms from which it may originate has previously been noted. PLK1 activity accumulates inversely to G2 checkpoint signal Current models propose that pro-mitotic activity is switched off during G2 checkpoint activation, and reactivated when checkpoint signalling falls below a defined threshold [19] . For instance, the activity of an essential pro-mitotic enzyme, PLK1, is reported to be extinguished by G2 checkpoint activation [21] , [23] , [49] , and its reactivation is thought necessary for recovery from G2 arrest [29] . This prompted us to investigate the correlation between pro-mitotic PLK1 activity and the observed heterogeneity in residual G2 checkpoint activation in cells recovering from G2 arrest. To do this, we simultaneously monitored the G2 checkpoint activation signal and PLK1 substrate phosphorylation in single living cells, by constructing a cell line that harbours mCherry-tagged MDC1 ( Supplementary Fig. 2A and B ), as well as a G2-specific PLK1 sensor [50] based on Förster resonance energy transfer (FRET), integrated into the genome ( Supplementary Fig. 2B ). The sensor contains a PLK1-specific phospho-epitope [50] , whose modification provides a measure of PLK1 substrate phosphorylation over time net of de-phosphorylation by competing phosphatases. As expected, PLK1 activity reported by the FRET sensor reflects phosphorylation of the endogenous PLK1 downstream substrate, Myt1 ( Supplementary Fig. 2C ) and peaks gradually during unperturbed G2/M progression ( Supplementary Fig. 2D ). To study the effect of damage-induced G2 checkpoint activation, single cells synchronized in G2 before exposure to a pulse of etoposide were imaged for 24 h to determine changes in the number of MDC1-mCherry foci and in relative PLK1 activity ( Fig. 3a , see Supplementary Methods ). Results were plotted for the cells that recovered from G2 arrest within this 24 h observation period, and for which images were available at each time-point from damage induction to mitotic entry. 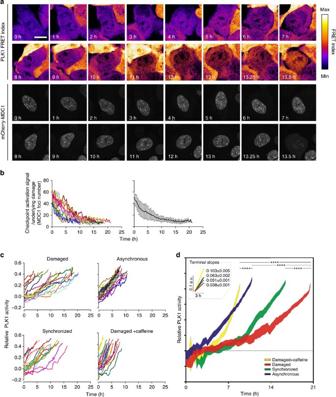Figure 3: Dynamics of damage repair and PLK1 activity from single-cell measurements. (a) Serial imaging of U2OS cells expressing the PLK1 sensor and MDC1-mCherry. U2OS cells synchronized in G2 were pulsed with etoposide as before and tracked by live cell imaging until just before NEBD at mitotic entry as described inFig. 2b. The images were analysed using custom-written MATLAB software to measure the nuclear PLK1 FRET index and MDC1 foci number at different time points. Scale bar, 5 μm. (b) Changes in the checkpoint activation signal (MDC1 foci number) in single cells (left) or on average (right) from the time of damage treatment until just before NEBD at mitotic entry (n=20). The coloured lines represent the trajectories of individual cells, and the single black lines represent the population average, with the standard deviation for each data point (bars). (c) The relative PLK1 activity at each time point, measured using the FRET index as described in Methods, was tracked by live cell imaging under various experimental conditions. Plots marked ‘damage’ shows results on U2OS cells, treated as described inFig. 2a, followed from the time of damage treatment until mitotic entry (n=20); ‘asynchronous’, shows results on asynchronous U2OS cells followed from initial PLK1 activation until mitotic entry (n=19); ‘synchronized’, shows results on U2OS cells synchronized in G2 after thymidine release, followed until mitotic entry (n=20); ‘damaged+caffeine’, shows results from a similar experiment on U2OS cells synchronized in G2, pulsed with 10 μM etoposide for 8 min, and then left in caffeine during live cell imaging (n=25). The coloured lines represent the trajectories of individual cells. (d) Traces from individual cells exposed to different treatments described incwere synchronized at mitotic entry and averaged within the same treatment groups. The mean and standard error of the average trajectories are shown. ‘Terminal slopes’ depicted in the top-left corner display the linear regression of the last 3 h of the traces, with the very last time point excluded. Analysis of covariance shows that the slopes in the different treatment groups are significantly different from one another. (****P<0.0001). Figure 3: Dynamics of damage repair and PLK1 activity from single-cell measurements. ( a ) Serial imaging of U2OS cells expressing the PLK1 sensor and MDC1-mCherry. U2OS cells synchronized in G2 were pulsed with etoposide as before and tracked by live cell imaging until just before NEBD at mitotic entry as described in Fig. 2b . The images were analysed using custom-written MATLAB software to measure the nuclear PLK1 FRET index and MDC1 foci number at different time points. Scale bar, 5 μm. ( b ) Changes in the checkpoint activation signal (MDC1 foci number) in single cells (left) or on average (right) from the time of damage treatment until just before NEBD at mitotic entry ( n =20). The coloured lines represent the trajectories of individual cells, and the single black lines represent the population average, with the standard deviation for each data point (bars). ( c ) The relative PLK1 activity at each time point, measured using the FRET index as described in Methods, was tracked by live cell imaging under various experimental conditions. Plots marked ‘damage’ shows results on U2OS cells, treated as described in Fig. 2a , followed from the time of damage treatment until mitotic entry ( n =20); ‘asynchronous’, shows results on asynchronous U2OS cells followed from initial PLK1 activation until mitotic entry ( n =19); ‘synchronized’, shows results on U2OS cells synchronized in G2 after thymidine release, followed until mitotic entry ( n =20); ‘damaged+caffeine’, shows results from a similar experiment on U2OS cells synchronized in G2, pulsed with 10 μM etoposide for 8 min, and then left in caffeine during live cell imaging ( n =25). The coloured lines represent the trajectories of individual cells. ( d ) Traces from individual cells exposed to different treatments described in c were synchronized at mitotic entry and averaged within the same treatment groups. The mean and standard error of the average trajectories are shown. ‘Terminal slopes’ depicted in the top-left corner display the linear regression of the last 3 h of the traces, with the very last time point excluded. Analysis of covariance shows that the slopes in the different treatment groups are significantly different from one another. (**** P <0.0001). Full size image The levels of the checkpoint activation signal in single cells monitored by the MDC1-mCherry decreased over time consistent with the known kinetics of DSB repair measured in cell populations [51] . This is evident from the single cell and population trajectories shown in Fig. 3b . Unexpectedly, however, relative PLK1 activity monitored by the FRET sensor increased progressively throughout the period of G2 arrest ( Fig. 3c , damaged). This occurred even at the earliest time points when levels of the checkpoint signal were relatively high. However, the rate of increase in cumulative PLK1 activity, represented by the slope of the curves, was significantly lower in cells exposed to damage ( Fig. 3c,d , damaged) compared with undamaged cells in asynchronous division ( Fig. 3c,d , asynchronous) or in undamaged cells synchronously entering mitosis ( Fig. 3c,d , synchronized). Importantly, PLK1 activity increased at a higher rate when etoposide-damaged cells were treated with caffeine ( Fig. 3c,d , damaged+caffeine), an inhibitor of G2 checkpoint signalling [52] , suggesting that checkpoint activation suppresses the rate of increase in PLK1 activity, but does not extinguish it. These observations substantiate that changes in PLK1 activity represent a key element controlling G2 checkpoint recovery in individual cells from the same population. Next, we studied the relationship between the G2 checkpoint activation signal and PLK1 activity. Individual single-cell trajectories ( Fig. 4a–c ) can be clustered into three distinct groups that exhibit differences in the initial level of PLK1 activity at the beginning of the experiment. Group 1 ( n =15 cells, starting FRET index (FI) >0.08 arbitrary units (a.u.)) entered mitosis relatively quickly in 5±1 h (mean±s.e.m) after DNA damage, and with a relatively high level of checkpoint activation signal represented by 15±2 foci (mean±s.e.m) at the time of mitotic entry. By contrast, cells in Group 2 ( n =12, starting FI=0–0.08 a.u.) entered mitosis slower in 13±2 h after DNA damage, accompanied by a low level of checkpoint activation signal represented by 9.9±0.9 foci. Finally, cells in Group 3 ( n =18, starting FI <0, that is, initial FI below the median value), which started with least PLK1 activity after DNA damage treatment, entered mitosis most slowly (14.4±0.9 h after damage) with a low level of checkpoint activation signal (8.0± 0.5 foci; Fig. 4d,e ). Notably, these results indicate that the variation in checkpoint activation signal at G2 recovery correlates with the initial level of PLK1 substrate phosphorylation ( Fig. 4a–c, e ), suggesting that the relative activity of PLK1 may determine the sensitivity of G2 arrest. 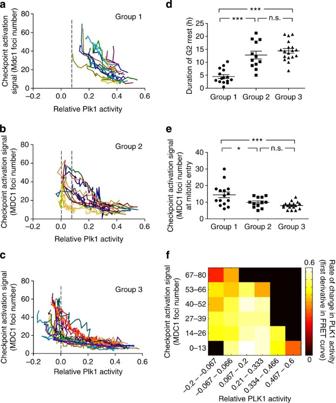Figure 4: Relationship between the level of checkpoint activation signal (MDC1 foci) and PLK1 activity. (a–c) U2OS cells expressing the PLK1 sensor and MDC1-mCherry were treated as inFig. 2aand tracked by live cell imaging until just before NEBD at mitotic entry as described inFig. 2b(n=45). Each coloured line represents the checkpoint activation signal (MDC1 foci) plotted against relative PLK1 activity in a single cell. Cells were categorized into three groups based on the initial value of the PLK1 activity. (a) Group 1: initial PLK1 activity >0.08; (b) Group 2: initial PLK1 activity between 0 and 0.08; (c) Group 3: initial PLK1 activity <0. (d) The duration of G2 arrest from DNA damage until mitotic entry in the three groups of cells showing the mean±s.e.m. Statistical analysis using analysis of variance (ANOVA)/Bonferroni test is displayed. The three groups are significantly different atP<0.0001. (e) The level of remaining checkpoint activation signal (MDC1 foci number) just before NEBD at mitotic entry in the three groups of cells, showing the mean±s.e.m. Statistical analysis using ANOVA/Bonferroni test is displayed. The three groups are significantly different atP<0.0001. (f) The rate of change in PLK1 activity (the first derivative of PLK1 activity over time) from single-cell measurements, represented by the colour map shown at the right, was plotted against the corresponding checkpoint activation signal (MDC1 foci number) on the vertical axis, and the relative change in PLK1 activity on the horizontal. Each box represents the average rate of changes in PLK1 activity in cells that fall within the corresponding range. NS, not significant. Figure 4: Relationship between the level of checkpoint activation signal (MDC1 foci) and PLK1 activity. ( a – c ) U2OS cells expressing the PLK1 sensor and MDC1-mCherry were treated as in Fig. 2a and tracked by live cell imaging until just before NEBD at mitotic entry as described in Fig. 2b ( n =45). Each coloured line represents the checkpoint activation signal (MDC1 foci) plotted against relative PLK1 activity in a single cell. Cells were categorized into three groups based on the initial value of the PLK1 activity. ( a ) Group 1: initial PLK1 activity >0.08; ( b ) Group 2: initial PLK1 activity between 0 and 0.08; ( c ) Group 3: initial PLK1 activity <0. ( d ) The duration of G2 arrest from DNA damage until mitotic entry in the three groups of cells showing the mean±s.e.m. Statistical analysis using analysis of variance (ANOVA)/Bonferroni test is displayed. The three groups are significantly different at P <0.0001. ( e ) The level of remaining checkpoint activation signal (MDC1 foci number) just before NEBD at mitotic entry in the three groups of cells, showing the mean±s.e.m. Statistical analysis using ANOVA/Bonferroni test is displayed. The three groups are significantly different at P <0.0001. ( f ) The rate of change in PLK1 activity (the first derivative of PLK1 activity over time) from single-cell measurements, represented by the colour map shown at the right, was plotted against the corresponding checkpoint activation signal (MDC1 foci number) on the vertical axis, and the relative change in PLK1 activity on the horizontal. Each box represents the average rate of changes in PLK1 activity in cells that fall within the corresponding range. NS, not significant. Full size image The heatmap in Fig. 4f plots the rate of increase in PLK1 activity (pseudo-coloured from white (high) to red (low)) against relative PLK1 activity (FI), and checkpoint activation signal. This analysis reveals that the rate of increase in PLK1 activity was higher in cells where relative PLK1 activity was also high (white or yellow boxes in Fig. 4f ), despite similar levels of the checkpoint activation signal. This suggests that cells with a higher existing level of PLK1 activity are less sensitive to the mitotic inhibitory effect of damage-induced G2 checkpoint activation. A threshold of cumulative PLK1 activity gates mitotic entry Interestingly, in all experimental conditions examined, G2 checkpoint recovery and entry into mitosis occur when cumulative PLK1 activity from the baseline until mitotic entry monitored by the FRET sensor approaches a FI value of ~0.4 a.u. (compare across Fig. 3c ). This value is independent of either the initial level of checkpoint activation signal/underlying damage (F test, P =0.5, range: 13–66 foci, Fig. 5a ) or the initial level of PLK1 activity ( P =0.6, range: from −0.08 to 0.37 a.u., Fig. 5b ). In contrast, the level of checkpoint activation signal represented by MDC1 foci at mitotic entry exhibits a positive correlation with the initial level of DNA damage (F test, P =0.008, Supplementary Fig. 3A ). Moreover, the mean cumulative PLK1 activity at mitotic entry is independent of DNA damage, cell-cycle synchronicity or checkpoint inhibition using caffeine ( Fig. 5c ), whereas the mean level of checkpoint activation signal at mitotic entry varies considerably between different experimental conditions ( Fig. 2e and Supplementary Fig. 3A ). These findings suggest that G2 checkpoint recovery occurs when cumulative phosphorylation of PLK1 substrates exceeds a set threshold, promoted by low levels of PLK1 activity during G2 even in the presence of DNA damage. A further line of evidence also supports this conclusion. Cells that failed to undergo checkpoint recovery and remain in G2 arrest during 24 h of observation after etoposide-induced damage consistently exhibited cumulative PLK1 activity less than the threshold ( Supplementary Fig. 3C ), even when their level of checkpoint activation signal was considerably lower than in cells that recovered from the checkpoint and entered mitosis ( Supplementary Fig. 3B ). 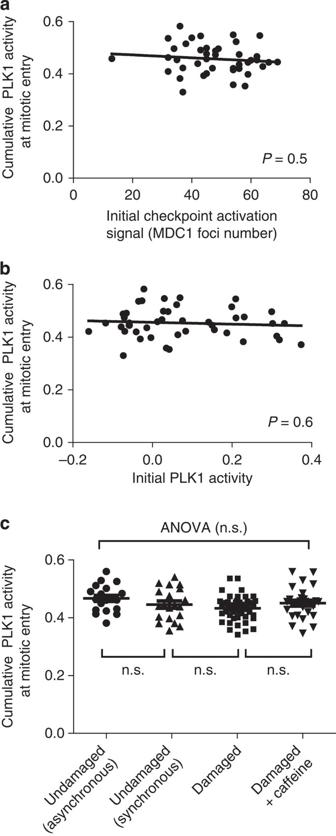Figure 5: A threshold for cumulative PLK1 activity gates mitotic entry. (a) For single cells, cumulative PLK1 activity at mitotic entry (change in the FRET index from the baseline) was plotted against the initial level of checkpoint activation signal (MDC1 foci number). The slope of the correlation between these two parameters did not differ significantly from zero (F test,P=0.5). (b) For single cells, cumulative PLK1 activity at mitotic entry (change in the FRET index from the baseline) was also plotted against the initial level of PLK1 activity. Again, the slope of the correlation between these two parameters did not differ significantly from zero (F test,P=0.6). (c) Cumulative PLK1 activity at mitotic entry (change in the FRET index from the baseline) was derived from the experimental data shown inFig. 3cfor cells exposed to different conditions. This graph compares cumulative PLK1 activity at mitotic entry in: asynchronous U2OS cells entering mitosis (undamaged (asynchronous)); cells synchronized in G2 after thymidine release (undamaged (synchronous); cells synchronized in G2 then exposed to DNA damage, without (damage) or with (damage+caffeine) caffeine treatment. In all these experimental conditions, there was no statistically significant difference (P>0.05) in cumulative PLK1 activity at mitotic entry using two different tests (analysis of variance (ANOVA) test, top,P=0.07; unpairedt-test, bottom,P=0.2, 0.3, 0.12 from left to right) . NS, not significant. Figure 5: A threshold for cumulative PLK1 activity gates mitotic entry. ( a ) For single cells, cumulative PLK1 activity at mitotic entry (change in the FRET index from the baseline) was plotted against the initial level of checkpoint activation signal (MDC1 foci number). The slope of the correlation between these two parameters did not differ significantly from zero (F test, P =0.5). ( b ) For single cells, cumulative PLK1 activity at mitotic entry (change in the FRET index from the baseline) was also plotted against the initial level of PLK1 activity. Again, the slope of the correlation between these two parameters did not differ significantly from zero (F test, P =0.6). ( c ) Cumulative PLK1 activity at mitotic entry (change in the FRET index from the baseline) was derived from the experimental data shown in Fig. 3c for cells exposed to different conditions. This graph compares cumulative PLK1 activity at mitotic entry in: asynchronous U2OS cells entering mitosis (undamaged (asynchronous)); cells synchronized in G2 after thymidine release (undamaged (synchronous); cells synchronized in G2 then exposed to DNA damage, without (damage) or with (damage+caffeine) caffeine treatment. In all these experimental conditions, there was no statistically significant difference ( P >0.05) in cumulative PLK1 activity at mitotic entry using two different tests (analysis of variance (ANOVA) test, top, P =0.07; unpaired t -test, bottom, P =0.2, 0.3, 0.12 from left to right) . NS, not significant. Full size image Furthermore, similar results were obtained from experiments in hTERT-RPE1 cells ( Supplementary Fig. 4 ). Thus, PLK1 activity exhibited similar kinetics, and continued to accumulate after exposure to 1 Gy IR, with a slower rate of increase than in undamaged cells (compare Supplementary Fig. 4A, B ), and cumulative PLK1 activity at mitotic entry reached a threshold value that was constant in the presence or absence of DNA damage ( Supplementary Fig. 4C ). These findings suggest that our conclusions are unlikely to be cell type specific. The mechanism we propose would permit the eventual escape from G2 of arrested cells that do not succumb to other outcomes (for example, apoptosis or senescence) even in the presence of DNA damage. Such a model predicts that a downstream effector of PLK1, like Cyclin B1, the synthesis of which is reported to be downstream of PLK1 activity [53] , would follow with its expression levels trajectories similar to those of PLK1 substrate phosphorylation. Indeed, the level of endogenous Cyclin B1 expression indeed exhibited patterns similar to those of PLK1 activity both in undamaged ( Supplementary Fig. 5A ) or DNA-damaged cells ( Supplementary Fig. 5B ). Moreover, the intracellular levels of Cyclin B1 also manifested a threshold value at mitotic entry, reminiscent of the observed threshold of PLK1 activity at the same juncture ( Supplementary Fig. 4C ). Finally, Cyclin B1 expression was well correlated with PLK1 activity measured by the FRET sensor over time ( Supplementary Fig. 5D ). Collectively, these results concerning endogenous Cyclin B1 expression provide further support for our conclusion that mitotic entry is triggered when cumulative PLK1 activity reaches a defined threshold, and suggest that Cyclin B1 may serve as a downstream effector of PLK1. Thus in summary, our findings suggest that G2 checkpoint recovery occurs when cumulative PLK1 activity approaches a set threshold that gates mitotic entry, regardless of the remaining checkpoint activation signal, DNA damage or the duration of G2 arrest. This predicts that experimentally induced alterations in PLK1 activity should concomitantly alter the characteristics of G2 checkpoint recovery. Manipulating PLK1 activity alters cell fate during recovery We therefore examined checkpoint recovery in cells synchronized in G2 that were treated with a specific small-molecule inhibitor of PLK1, BI2536 (ref. 54 ), following exposure to a pulse of etoposide, as previously described. BI2536 exposure not only markedly suppressed relative PLK1 activity measured by the FRET sensor in undamaged cells ( Supplementary Fig. 6 ), but also sharply inhibited any increase in PLK1 activity over time in G2-arrested cells exposed to DNA damage ( Fig. 6a ). As expected, only 2 of 34 BI2536-treated cells (<6%) entered mitosis during the 24 h observation period following etoposide treatment ( Fig. 6b ), as compared with around 50% of cells not exposed to the inhibitor. The level of the checkpoint activation signal represented by MDC1 foci number in BI2536-treated cells that remain in G2 was considerably lower ( Supplementary Fig. 3B ) than in cells that entered mitosis in the absence of BI2536, consistent with the idea that cumulative PLK1 activity rather than the amount of remaining checkpoint activation signal determines mitotic entry. 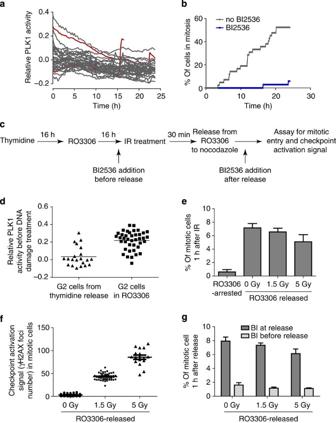Figure 6: PLK1 activity as a determinant of G2 checkpoint recovery. (a) U2OS cells synchronized in G2 were pulsed with etoposide and treated with PLK1 inhibitor, BI2536, during live cell imaging. The trajectories represent the relative PLK1 activity for single cells. Grey lines represent the trajectories of individual cells not entering mitosis over the period of observation (n=32), whereas the red lines represent two cells that entered. (b) Kinetics of mitotic entry in U2OS cells after DNA damage during G2, with or without BI2536 treatment. The cumulative percentage of mitotic entry over 24 h is shown. (c) The experimental protocol for the experiments inb,d–f. Cells were released from thymidine into medium containing Cdk1 inhibitor, RO3306, for 16 h until progression into G2. Cells were then treated with different doses of IR (0, 1.5 or 5 Gy). After 30 min, cells were released from RO3306 into nocodazole-containing medium to trap cells that recovered from G2 arrest. BI2536 was added to inhibit PLK1 activity either at the time of release from RO3306 or 5 h before release. (d) U2OS cells were synchronized in G2 by allowing progression for 7.5 h after thymidine release (G2 cells, thymidine release) or by treatment with RO3306 for 16 h after thymidine release (G2 cells, RO3306) and then exposed to DNA damage. Relative PLK1 activity in single cells before DNA damage in both conditions is shown in the dot plot. (e) The percentage of MPM2-positive mitotic cells 1 h after release from RO3306 (RO3306-released) after exposure to different doses of IR is shown. The first bar shows the results from cells left in RO3306-containing medium (RO3306-arrested) as control. (f) The level of checkpoint activation signal (marked by γH2AX foci number) in cells that escaped from G2 arrest and entered mitosis within 1 h after release from RO3306 is shown. (g) The percentage of MPM2-positive mitotic cells 1 h after release from RO3306 after different doses of IR treatment is shown. BI2536 was added at the time of release from RO3306 (black bars), or 5 h before release (grey bars), to inhibit PLK1 activity. Figure 6: PLK1 activity as a determinant of G2 checkpoint recovery. ( a ) U2OS cells synchronized in G2 were pulsed with etoposide and treated with PLK1 inhibitor, BI2536, during live cell imaging. The trajectories represent the relative PLK1 activity for single cells. Grey lines represent the trajectories of individual cells not entering mitosis over the period of observation ( n =32), whereas the red lines represent two cells that entered. ( b ) Kinetics of mitotic entry in U2OS cells after DNA damage during G2, with or without BI2536 treatment. The cumulative percentage of mitotic entry over 24 h is shown. ( c ) The experimental protocol for the experiments in b , d – f . Cells were released from thymidine into medium containing Cdk1 inhibitor, RO3306, for 16 h until progression into G2. Cells were then treated with different doses of IR (0, 1.5 or 5 Gy). After 30 min, cells were released from RO3306 into nocodazole-containing medium to trap cells that recovered from G2 arrest. BI2536 was added to inhibit PLK1 activity either at the time of release from RO3306 or 5 h before release. ( d ) U2OS cells were synchronized in G2 by allowing progression for 7.5 h after thymidine release (G2 cells, thymidine release) or by treatment with RO3306 for 16 h after thymidine release (G2 cells, RO3306) and then exposed to DNA damage. Relative PLK1 activity in single cells before DNA damage in both conditions is shown in the dot plot. ( e ) The percentage of MPM2-positive mitotic cells 1 h after release from RO3306 (RO3306-released) after exposure to different doses of IR is shown. The first bar shows the results from cells left in RO3306-containing medium (RO3306-arrested) as control. ( f ) The level of checkpoint activation signal (marked by γH2AX foci number) in cells that escaped from G2 arrest and entered mitosis within 1 h after release from RO3306 is shown. ( g ) The percentage of MPM2-positive mitotic cells 1 h after release from RO3306 after different doses of IR treatment is shown. BI2536 was added at the time of release from RO3306 (black bars), or 5 h before release (grey bars), to inhibit PLK1 activity. Full size image Next, we elevated PLK1 activity before the exposure of cells to DNA damage to test whether G2 checkpoint recovery would occur more quickly. Cells can be arrested late in the G2 phase ( Fig. 6c ) if treated with the CDK1-specific small-molecule inhibitor RO3306 (ref. 55 ) for 16 h after thymidine release. A majority of the cells synchronized in this way exhibited a higher level of PLK1 FRET sensor phosphorylation as compared with cells synchronized in G2 after thymidine release ( Fig. 6d ). We then exposed RO3306-synchronized cells to different doses of IR, and 30 min afterwards, released them from RO3306 into nocodazole-containing medium to trap cells that recovered from G2 arrest to enter mitosis ( Fig. 6c ). Notably, RO3306-synchronized cells exposed to DNA damage very quickly recovered from G2 arrest similar to undamaged cells, with ~7% of cells in both experimental conditions entering mitosis by 1 h ( Fig. 6e ). Moreover, these cells entering mitosis 1 h after 1.5 Gy IR treatment exhibited a relatively high average level of checkpoint activation signal represented by γH2AX foci (mean=43±6 foci per cell, Fig. 6f ). RO3306-synchronized cells exposed to a higher dose (5 Gy) of DNA damage also recovered quickly from G2 checkpoint arrest, with 5% entering mitosis within 1 h ( Fig. 6e ), still containing very high levels of checkpoint activation signal (mean=85±18 foci per cell, Fig. 6f ). Thus, collectively, our experiments using chemical inhibitors to experimentally manipulate the PLK1 kinase support the conclusion that G2 checkpoint recovery occurs heterogeneously in single cells via a mechanism dependent on cumulative PLK1 activity that gates mitotic entry at a defined threshold. Experiments presented earlier in this report also speak to the same conclusion. Thus, Group 1 cells with a high initial level of PLK1 activity continue to accumulate PLK1 substrate phosphorylation relatively swiftly after DNA damage ( Fig. 4a ), recovering from G2 arrest and entering mitosis within a short period ( Fig. 4d ), even though they retain a relatively high level of the checkpoint activation signal ( Fig. 4e ). Interestingly, the entry into mitosis of cells synchronized in late G2 by RO3306 treatment was sharply suppressed when the PLK1 inhibitor BI2536 was added before DNA damage but not when BI2536 was added after release from RO3306 ( Fig. 6c,g ). This observation suggests that cumulative PLK1 activity over the period in damage-induced G2 arrest, rather than the transient levels after damage, determine checkpoint recovery and entry into mitosis. Our findings suggest a homeostatic mechanism for the G2 checkpoint in human cells wherein its outcome is determined by a dynamic balance between opposing signals for checkpoint activation and pro-mitotic activities that is represented (integrated) by cumulative PLK1 activity ( Fig. 7 ). Thus, individual cells from the same population recover from checkpoint activation to enter mitosis after varying durations of arrest, and with different levels of remaining checkpoint signal or DNA damage. This non-genetic heterogeneity is controlled via changes in the rate of accumulation of PLK1 activity in each cell. PLK1 activity continues to accumulate from its initial level in each G2-arrested cell, inversely correlated with the strength of the checkpoint activation signal elicited by DNA damage, until it reaches a threshold sufficient to trigger mitotic entry. As a result, cell-to-cell heterogeneity in the outcome of G2 arrest is dependent on variables such as the initial level of DNA damage, or the pre-existing level of PLK1 activity before damage imposition ( Supplementary Fig. 3A and Fig. 4a–e ). In such a mechanism, cumulative PLK1 activity represents a key element of an interaction loop, triggering a change in state from G2 arrest to mitotic entry when it exceeds a critical gating value ( Fig. 7 ). 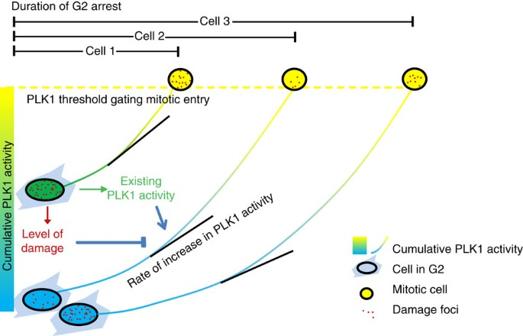Figure 7: Hypothetical model for homeostatic control of the G2 checkpoint in human cells. Key features of a hypothetical model for homeostatic control of the G2 checkpoint are schematically illustrated. During G2 arrest induced by DNA damage, cells continue to accumulate PLK1 activity (left) until its cumulative value reaches a threshold (yellow dotted line, top) that gates mitotic entry. Note that G2-arrested cells may have different initial levels of existing PLK1 activity (compare cells at left). The rate of increase in PLK1 activity (black lines, centre) in any given cell is negatively correlated to the level of DNA damage (red dots in cell nuclei) but positively correlated to existing level of PLK1 activity. The integration of these parameters determines the duration of G2 arrest, and the amount of DNA damage or checkpoint activation signal in mitotic cells that have recovered from G2 arrest (lines at the top). The comparison between cells 1 and 3 illustrates the effect of levels of initial PLK1 activity on the duration of G2 arrest. Thus, cell 1, which arrests with a high level of initial PLK1 activity, exhibits a shorter duration of G2 arrest despite a high level of DNA damage. In contrast, cell 3, which arrests with a low level of initial PLK1 activity, exhibits a longer duration of G2 arrest despite bearing the same level of DNA damage as cell 1, and enters mitosis with a lower number of damage foci owing to the increased time for G2 repair. The comparison between cells 2 and 3 illustrates the effect of different amounts of DNA damage on the rate of accumulation of PLK1 activity and the duration of mitotic arrest. Thus, cells 2 and 3 arrest with similar low levels of PLK1 activity. However, the rate of accumulation of PLK1 activity is higher in cell 2 than in cell 3 because it bears a lower amount of DNA damage, and so cell 2 recovers from the G2 checkpoint and enters mitosis more quickly than cell 3, and with a different amount of residual checkpoint signal or underlying DNA damage. Figure 7: Hypothetical model for homeostatic control of the G2 checkpoint in human cells. Key features of a hypothetical model for homeostatic control of the G2 checkpoint are schematically illustrated. During G2 arrest induced by DNA damage, cells continue to accumulate PLK1 activity (left) until its cumulative value reaches a threshold (yellow dotted line, top) that gates mitotic entry. Note that G2-arrested cells may have different initial levels of existing PLK1 activity (compare cells at left). The rate of increase in PLK1 activity (black lines, centre) in any given cell is negatively correlated to the level of DNA damage (red dots in cell nuclei) but positively correlated to existing level of PLK1 activity. The integration of these parameters determines the duration of G2 arrest, and the amount of DNA damage or checkpoint activation signal in mitotic cells that have recovered from G2 arrest (lines at the top). The comparison between cells 1 and 3 illustrates the effect of levels of initial PLK1 activity on the duration of G2 arrest. Thus, cell 1, which arrests with a high level of initial PLK1 activity, exhibits a shorter duration of G2 arrest despite a high level of DNA damage. In contrast, cell 3, which arrests with a low level of initial PLK1 activity, exhibits a longer duration of G2 arrest despite bearing the same level of DNA damage as cell 1, and enters mitosis with a lower number of damage foci owing to the increased time for G2 repair. The comparison between cells 2 and 3 illustrates the effect of different amounts of DNA damage on the rate of accumulation of PLK1 activity and the duration of mitotic arrest. Thus, cells 2 and 3 arrest with similar low levels of PLK1 activity. However, the rate of accumulation of PLK1 activity is higher in cell 2 than in cell 3 because it bears a lower amount of DNA damage, and so cell 2 recovers from the G2 checkpoint and enters mitosis more quickly than cell 3, and with a different amount of residual checkpoint signal or underlying DNA damage. Full size image In contrast to previous studies focusing on populations rather than single cells [19] , our single-cell quantitative measurements are inconsistent with the idea that G2 checkpoint activation by DNA damage arrests mitotic entry until DNA repair allows checkpoint signalling to fall below a defined threshold. Our results are also at odds with the proposal, again originating from ensemble studies, that checkpoint signalling acts as an ‘on-off’ switch to extinguish pro-mitotic signals like PLK1 activity. Instead, we observe a wide heterogeneity in residual checkpoint activation signal or underlying DNA damage at mitotic entry in single cells, which appears to be the manifestation of the progressive accumulation of PLK1 activity at different rates in each cell that occurs even in the presence of checkpoint activation. Thus, our studies exemplify the power of single-cell quantitative analyses to reveal cell-to-cell variations that provide fresh insight into the mechanisms governing cell fate during recovery from G2 checkpoint arrest. Cumulative PLK1 substrate phosphorylation monitored by the FRET sensor used in our work is likely to reflect a collective pro-mitotic potential to activate CDK1, because PLK1 directly phosphorylates many substrates during G2 that contribute directly to CDK1 activation, including Myt1 and Cdc25C [56] , [57] . Thus, our observation that G2 checkpoint recovery and mitotic entry occur when cumulative PLK1 activity exceeds a set value may reflect an underlying threshold of PLK1 substrate phosphorylation necessary for the bi-stable activation of CDK1. Indeed, we find that endogenous Cyclin B1, the activator of CDK1 whose transcription depends on PLK1 activity, also continuously accumulated during DNA damage-induced G2 arrest until it reached a threshold level during checkpoint recovery, akin to the observed changes in PLK1 activity. On the other hand, the inhibition of PLK1 kinase activity delays but does not prevent CDK1 activation [29] , [58] , raising the possibility that redundant pro-mitotic activities fostering CDK1 activation (such as Aurora A activity) may behave in a similar manner to PLK1 during G2 checkpoint recovery. It will be interesting in future studies to test this possibility. Nevertheless, the findings we report here clearly show that cumulative PLK1 activity monitored by the FRET sensor correlates with the potential for G2 checkpoint recovery and mitotic entry. Thus, variation in the initial level of PLK1 substrate phosphorylation directly contributes to the probability that cells enter mitosis with varying levels of checkpoint activation signal ( Fig. 4a–e ). Moreover, experimentally induced alterations in PLK1 activity predictably alter the levels of checkpoint activation signal or DNA damage tolerated at mitotic entry ( Fig. 6 ). Our findings concerning the mechanism of G2 checkpoint recovery provoke comparisons with the mitotic spindle assembly checkpoint (SAC). We find that cumulative PLK1 activity progressively accumulates even in the face of an active checkpoint signal or underlying DNA damage, but at a rate inversely correlated to the strength of this parameter, and thereby serves to integrate these opposing pro-mitotic versus anti-mitotic signals. This is reminiscent of findings concerning mitotic slippage after SAC arrest. During cell-cycle arrest at the SAC because of improperly attached kinetochores, the checkpoint signal is progressively opposed by the gradual degradation of Cyclin B1 via the decreased but not absent activity of the anaphase-promoting complex/cyclosome (APC/C), to allow mitotic slippage [59] , [60] . In turn, the activity of the APC/C is homeostatically controlled by opposing checkpoint-sustaining and -repressing forces that regulate the levels of its essential co-factor, Cdc20 (refs 61 , 62 ). Our findings suggest, however, that G2 checkpoint recovery despite persistent underlying DNA damage may occur more readily than mitotic slippage despite incomplete kinetochore-microtubule attachment. This may be related to the kinetics of the opposing events—thus, both DNA repair and the progressive accumulation of PLK1 activity occur over periods spanning minutes to hours, but kinetochore attachment can occur in minutes, whereas gradual Cyclin B1 degradation when the SAC is active takes hours. One corollary of this suggestion is that the level of PLK1 activity may be critical in determining whether or not cells tolerate cell division despite persistent DNA damage, which may be of particular importance during oncogenic transformation, or the response of cancer cells to DNA-damaging agents. Thus, a homeostatic mechanism for the G2 checkpoint wherein checkpoint recovery is heterogeneously determined in each single cell by the integration of different pathways into cumulative PLK1 activity has implications for cancer pathogenesis and treatment that warrant future investigation. Cell culture and synchronization U2OS cells (European Collection of Cell Cultures) were grown in standard DMEM supplemented with 10% FCS. hTERT-RPE1 cells were grown in F12/DMEM (1:1) supplemented with 10% FCS. Cells were maintained at 37 °C with 5% CO 2 . Cells were grown on plastic dishes for maintenance and on poly- D -lysine-coated 35 mm glass bottom dishes No. 1.0 MatTek chamber for live cell imaging. To synchronize cells in early S phase, 2 mM thymidine was added to cultures (at a confluency of 50–70%) for 16 h. Cells were either released from thymidine for subsequent assays or treated with thymidine again for 8 h before release for ‘double thymidine synchronization’. Immunoprecipitation and western blotting Cells harvested by trypsinization were lysed in RIPA buffer and incubated with anti-GFP (Living Colors A.V., 1:1,000) primary antibody and anti-mouse IgG-conjugated beads overnight at 4 °C. Immunoprecipitates or whole protein lysates were separated by electrophoresis and transferred to polyvinylidene difluoride membranes, which were blocked in 5% skim milk dissolved in Tris-buffered saline (TBS)-Tween and incubated with a primary antibody (anti-mCherry (Novus Biological (NBP1-96752), 1:1,000), anti-Hsp90 (Cell Signaling (4877-1:5,000), 1:5,000), anti-Mdc1 (Abcam (ab11169), 1:1,000) or anti-phospho-threonine (Cell Signaling (9381), 1:1,000)) followed by anti-mouse IR800 CW or IR680 RD (Li-Cor, 1:5,000) secondary antibody. Membranes were scanned using an Odyssey infrared imaging system (LI-COR). FACS staining Trypsinized cells were fixed in 4% paraformaldehyde followed by 70% ethanol at −20 °C. Cells were incubated in blocking solution (PBS with 0.2% Triton X-100, 1% BSA) and subsequently incubated in anti-phospho-histone H3 primary antibody (Millipore (06–570), 1:500) or anti-MPM2 antibody (Millipore (05–368), 1:500) followed by secondary antibody conjugated with Alexa-488 (Life Technology, 1:500). DNA was stained with 40 μg ml −1 propidium iodide solution. Cytospin and immunofluorescence staining 1 × 10 5 harvested cells were loaded onto a cytofunnel aligned with polysine slides. The cells were settled onto slides by spinning at 800 r.p.m. for 3 min. Subsequently, cells were fixed by 4% paraformaldehyde solution. Cells were then permeabilized in 0.5% Triton X-100/TBS and blocked in 2% BSA, 0.1% Triton X-100/TBS solution. Primary antibodies were incubated at room temperature (RT) for 2 h (anti-γH2AX (Millipore (05–636), 1:2,000), anti-pH3 (Millipore, 1:1,000), anti-pS1981 ATM (Cell Signaling (4526), 1:1,000) or anti-Cyclin B1 (Santa Cruz (sc-245), 1:1,000)) followed by an appropriate secondary antibody conjugated to Alexa fluorophores (Life Technology, 1:500) for 1 h at RT. Cells were mounting with Vectashield containing 4',6-diamidino-2-phenylindole (DAPI). Metaphase spread and chromatin staining Cells were treated with Colcemid for 1.5 h before harvesting by trypsinization, incubation with hypotonic solution (1:1 of 0.4% KCl/0.4% sodium citrate) for 30 min at RT, and fixation in three changes of 3:1 MeOH to acetic acid. Cells were dropped onto pre-cleaned slides and allowed to dry overnight. Slides were stained and mounted with Vectashield containing DAPI. Image acquisition and analysis for fixed samples To analyse mitotic γH2AX foci, stained cells were imaged on a Leica SP5 confocal microscope (Leica) with pinhole equivalent to a 1.5-μm optical slice. A stack of eight optical slices was acquired at 1.5 μm step size for each field. Maximum projections of confocal image stacks were generated and analysed with Cellomics Bioapplications software using the Compartment Analysis 4 (Thermo Scientific) algorithm for nuclei segmentation (based on nuclear DAPI staining) and nuclear foci counts (γH2AX staining) in mitotic cells (with pH3 intensity above a set threshold). The thresholds for segmentation and foci counts were optimized for each independent experiment but were kept constant for different samples within one experiment. The results of this unsupervised procedure were manually checked. Average foci number and percentage of mitotic cells at each time point were plotted against one another in a ‘fate diagram’ as described in the text. Live cell imaging and imaging processing by MATLAB The PLK1 sensor plasmid was from Professor Michael Lampson (University of Pennsylvania, Philadelphia), and the MDC1-mCherry plasmid was cloned from a MDC1-GFP construct supplied by Dr Jiri Lukas. Cells were plated in MatTek chambers and synchronized in thymidine before releasing into cell cycle. After 6 h (RPE1) or 7.5 h (U2OS) release, DNA damage was induced with either IR at the indicated dose, or 10 μM etoposide pulse, as described in the text. The chamber was sealed with parafilm and the cells were maintained in CO 2 -independent Leibowitz’s L15 medium supplemented with 10% FCS. Cells were imaged using a Leica SP5 confocal microscope (Leica) enclosed in a 37 °C incubator, with a × 40 (numerical aperture=1.25) objective, × 3.5 digital zoom and pinhole equivalent to a 1.5-μm optical slice. Cyan fluorescent protein (CFP), GFP, yellow fluorescent protein (YFP) or mCherry were excited with the 458, 488, 513 or 594 nm laser lines, respectively. The laser power was adjusted to minimize photo-bleaching and photo-toxicity. A stack of eight optical slices was acquired at 1.5 μm step size for each field. Live cell imaging was started 40 min after DNA damage treatment and images were recorded every 15 min for up to 24 h. Custom software written in MATLAB (MathWorks) was used for analysis of live cell imaging data. For MDC1 detection, maximum projections of all z-stack images were generated and cell nuclei were segmented based on nuclear intensity of MDC1-mCherry after image smoothing. Foci were recognized by identifying the local maxima of MDC1 intensity detected over an auto-threshold generated by Otsu’s method in order to account for different backgrounds of MDC1 because of differential expression levels in cells. In some cases, manual counting was performed to validate the result from software counting. To extract the FI from the PLK1 sensor, nuclear intensity of CFP and YFP signals from all z-stacks was calculated. The ratio of CFP intensity over YFP intensity was calculated as the FI. To compare changes under different conditions, and data collected in different imaging sessions, the FI was normalized to the median value of initial FI computed over the population of cells imaged within an experiment. Changes in PLK1 activity over time were represented by the FI changes calculated as: where Δ E t is the standardized FI at time point ‘ t ’ and median(FI t=0 ) is the median value of the FI computed at the initial time point for all curves within an experimental session. Similarly, FRET changes at NEBD (Δ E ) are calculated as: where FI NEBD is the FI at the time of NEBD. A first-order correction of photo-bleaching for the FI was applied to avoid photo-bleaching-related artefacts. How to cite this article : Liang, H. et al . Homeostatic control of polo-like kinase-1 engenders non-genetic heterogeneity in G2 checkpoint fidelity and timing. Nat. Commun. 5:4048 doi: 10.1038/ncomms5048 (2014).